Identification of a genomic enhancer that enforces proper apoptosis induction in thymic negative selection 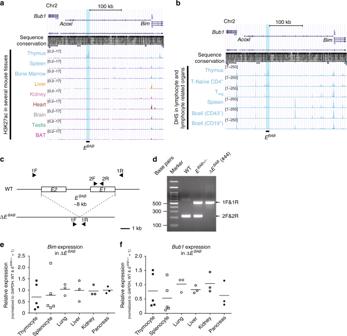Fig. 1 Identification of a T cell-specificcis-regulatory elementEBAB.aChIP-seq visualization of H3K27ac in several mouse tissues. H3K27ac profiles from the thymus, spleen, bone marrow, liver, kidney, heart, brain, testis, and brown adipose tissues (BAT) are visualized using the UCSC genome browser (mm9). TheEBABregion is highlighted.bDNase hypersensitivity sites (DHS) in the same locus shown in (a). DHS profiles from the thymus, T-Naïve CD4+, regulatory T (Treg) cells, spleen, and B cells (CD43−or CD19+) are visualized using the UCSC genome browser (mm9). TheEBABregion is highlighted.cSchematic representation of ΔEBAB. Arrowheads indicate the primers listed in Supplementary Data1.dGenomic PCR against theEBABlocus of WT, heterozygotes (EBAB+/−), and ΔEBABmice. A representative gel-image of founder #44-derived DNAs is shown. See also Supplementary Fig.2for the results from #47- and #50-derived DNAs.e,fqPCR analysis forBim(e) andBub1(f) on thymocytes, splenocytes, lung, liver, kidney, and pancreas. Data are pooled from five independent experiments (thymocyte, splenocyte;n= 5 WT andEBAB+/−–ΔEBABlittermate pairs, 7–17 weeks old, mean ± s.d.) or three independent experiments (lung, liver, kidney, pancreas;n= 3 WT &EBAB+/−–ΔEBABlittermate pairs, 10–17 weeks old). Each symbol represents an individual mouse; small horizontal lines indicate the mean. No statistically significant differences between WT andEBAB+/−and ΔEBABwere detected (P≥ 0.05; unpaired two-tailed Student’sttest) During thymic negative selection, autoreactive thymocytes carrying T cell receptor (TCR) with overtly strong affinity to self-MHC/self-peptide are removed by Bim-dependent apoptosis, but how Bim is specifically regulated to link TCR activation and apoptosis induction is unclear. Here we identify a murine T cell-specific genomic enhancer E BAB ( Bub1 - Acoxl - Bim ) , whose deletion leads to accumulation of thymocytes expressing high affinity TCRs. Consistently, E BAB knockout mice have defective negative selection and fail to delete autoreactive thymocytes in various settings, with this defect accompanied by reduced Bim expression and apoptosis induction. By contrast, E BAB is dispensable for maintaining peripheral T cell homeostasis via Bim-dependent pathways. Our data thus implicate E BAB as an important, developmental stage-specific regulator of Bim expression and apoptosis induction to enforce thymic negative selection and suppress autoimmunity. Our study unravels a part of genomic enhancer codes that underlie complex and context-dependent gene regulation in TCR signaling. T cell population in the thymus is highly heterogeneous, harboring a diverse T cell receptor (TCR) repertoire [1] , [2] , [3] , [4] . The massive diversity in TCR sequences is on one hand useful, as it puts the immune system on stand-by for numerous foreign antigens such as pathogens, while on the other hand it is risky because it could generate T cells harboring TCRs that strongly recognize self, potentially causing autoimmunity. To suppress autoimmunity, organisms have evolved a sophisticated mechanism called negative selection, establishing central T cell tolerance. In negative selection, interaction between TCR and self-peptide presented on major histocompatibility complexes (self-pMHCs) is converted into apoptotic output: high-affinity TCR clones are considered as autoreactive and die by apoptosis [1] , [2] , [3] , [4] . A part of high-affinity TCR clones, instead of being deleted, are diverted into regulatory T (T reg ) cells that are potent to suppress autoreactive T cells in periphery [1] , [5] . Suppression by T reg cells is one of the peripheral tolerance mechanisms for organisms to deal with autoreactive T cells that have evaded negative selection. Other mechanisms are induction of T cell anergy and peripheral deletion by apoptosis [1] . Pro-apoptotic Bim promotes the mitochondrial apoptosis cascade, contributing to numerous biological pathways [6] , [7] , [8] , [9] , [10] , [11] , [12] , [13] , [14] , [15] , [16] , [17] , [18] . In central T cell tolerance, Bim is considered as a downstream target of TCR signal: TCR signal activates Bim expression, and Bim knockout (KO) mice show defective negative selection [6] . However, little is known about how TCR signal strength is linked to Bim expression [2] , [17] . Bim is genetically required not only for establishing central T cell tolerance [6] , [7] , [8] , but also for depleting activated T cells in periphery [11] , [12] , B cell homeostasis, embryonic development, and so on [18] . Therefore, Bim should be able to distinguish multiple biological pathways in different cell types, depending on signals that cells receive. The molecular mechanism underlying how Bim is regulated to work at an appropriate place and time remains elusive. Enhancers are genomic elements that regulate gene expression in a signal and cell type dependent manner [19] , [20] . Although epigenome analyses have enabled systematic identification and characterization of enhancers, it is still difficult to directly study their physiological roles in vivo for the following reasons. First, enhancers are located often several hundreds of kilobases to even megabases away from their target genes, making it difficult to confidently predict a target(s) of an enhancer. Second, some genes may have multiple functionally redundant enhancers. Third, making enhancer KOs through genetic ablation has been labor-intensive and time-consuming, especially in mice. Recent progress in CRISPR–Cas9 technology [21] has reduced the cost and time needed for generating enhancer KO mice, and most importantly, has enabled us to produce large genomic deletions without leaving unwanted footprints of exogenous DNAs. CRISPR–Cas9 technology is indeed beginning to uncover physiological functions of novel enhancers in vivo [22] , [23] , [24] . Here, we utilize enhancer genetics to understand how Bim is specifically regulated to induce apoptosis during thymic negative selection, and find a cis -regulatory enhancer specifically contributing to this process. With the aid of epigenome analyses, we identify a cis -regulatory enhancer E BAB ( Bub1 - Acoxl - Bim ) that is specific to thymocytes and splenic T cells. We generate E BAB KO mice by CRISPR–Cas9 technology and find that a high-affinity TCR repertoire accumulates in the E BAB KO thymus. E BAB KO thymocytes are defective in apoptosis due to incomplete activation of Bim . By contrast, Bim -mediated homeostasis of T reg cells and peripheral T cells is not affected by E BAB KO, thereby implicating a specific function of E BAB in thymic negative selection. This study is an example of utilizing enhancer KO approach to dissect regulation of enhancer activity and subsequent gene function in vivo to address biological questions. Identification of a murine T cell-specific enhancer E BAB Our analyses on various publicly available ChIP-seq (chromatin-immunoprecipitation and following sequencing) data on multiple mouse tissues identified a T cell-specific enhancer-like region (H3K27ac high and H3K4me3 low) [19] in the mouse Bub1 - Acoxl - Bim locus (Fig. 1a and Supplementary Fig. 1 ). This region was located at approximately 200-kb upstream of Bim , within the ninth intron of Acoxl gene (unexpressed in T cells), and at approximately 90-kb upstream of Bub1 (a mitotic checkpoint factor), and thus was named E BAB . E BAB was approximately 8-kb in length and contained two prominent H3K27ac peaks E1 and E2 (Fig. 1a ). Both E1 and E2 were highly specific to the thymus (Fig. 1a ) and well conserved between human and mice (Fig. 1a and Supplementary Fig. 1b ). H3K27ac peaks corresponding to E BAB were identified also in the spleen to a lesser extent (Fig. 1a ). The signals in the spleen were likely derived from splenic peripheral T cells because naïve peripheral T cells, but not CD19 + B cells, retained DNase hypersensitivity sites in the locus (Fig. 1b ), the observation further supported by other publicly available ChIP-seq data sets (Supplementary Fig. 1c ). Fig. 1 Identification of a T cell-specific cis -regulatory element E BAB . a ChIP-seq visualization of H3K27ac in several mouse tissues. H3K27ac profiles from the thymus, spleen, bone marrow, liver, kidney, heart, brain, testis, and brown adipose tissues (BAT) are visualized using the UCSC genome browser (mm9). The E BAB region is highlighted. b DNase hypersensitivity sites (DHS) in the same locus shown in ( a ). DHS profiles from the thymus, T-Naïve CD4 + , regulatory T (T reg ) cells, spleen, and B cells (CD43 − or CD19 + ) are visualized using the UCSC genome browser (mm9). The E BAB region is highlighted. c Schematic representation of Δ E BAB . Arrowheads indicate the primers listed in Supplementary Data 1 . d Genomic PCR against the E BAB locus of WT, heterozygotes ( E BAB +/− ), and Δ E BAB mice. A representative gel-image of founder #44-derived DNAs is shown. See also Supplementary Fig. 2 for the results from #47- and #50-derived DNAs. e , f qPCR analysis for Bim ( e ) and Bub1 ( f ) on thymocytes, splenocytes, lung, liver, kidney, and pancreas. Data are pooled from five independent experiments (thymocyte, splenocyte; n = 5 WT and E BAB +/− –Δ E BAB littermate pairs, 7–17 weeks old, mean ± s.d.) or three independent experiments (lung, liver, kidney, pancreas; n = 3 WT & E BAB +/− –Δ E BAB littermate pairs, 10–17 weeks old). Each symbol represents an individual mouse; small horizontal lines indicate the mean. No statistically significant differences between WT and E BAB +/− and Δ E BAB were detected ( P ≥ 0.05; unpaired two-tailed Student’s t test) Full size image To investigate a physiological role of E BAB in vivo, we generated E BAB KO mice by using the CRISPR–Cas9 system (Fig. 1c and Supplementary Data 1 ). Three founder lines (line#44, #47 and #50) were successfully obtained, each harboring a distinct pattern of deletion (Fig. 1d and Supplementary Fig. 2 ). Because offspring from these different founders showed no phenotypic differences (Supplementary Fig. 3 ), we refer to these three KO alleles simply as Δ E BAB in this paper. To ask if E BAB KO affects expression of Bim and Bub1 , we performed quantitative polymerase chain reaction (qPCR) experiments on several organs and cell types including thymocytes and splenocytes (Fig. 1e, f ). Bim and Bub1 expression were slightly decreased in thymocytes and splenocytes in Δ E BAB mice (7–17 weeks old), while unaltered in the lung, liver, kidney, and pancreas (Fig. 1e, f ). Thus, E BAB is an enhancer specific to thymocytes and splenic T cells (Fig. 1a, b and Supplementary Fig. 1 ), deletion of which only slightly affected its proximal genes Bim and Bub1 in total thymocytes and splenocytes (Fig. 1e, f ). E BAB KO accumulates high-affinity TCR clones in the thymus Next, we asked whether Δ E BAB impairs T cell homeostasis in the thymus. For this purpose, thymocytes were analyzed using flow cytometry with anti-CD4 and anti-CD8 antibodies (Fig. 2a–d ). While the extent of reduction in Bim and Bub1 expression was very modest in Δ E BAB thymocytes (Fig. 1e, f ), severe abnormalities in thymocyte population were observed both in young (7–17 weeks old) and aged (30–36 weeks old) mice (Fig. 2a, b ): Δ E BAB increased proportion of double negative (DN), CD4 single positive (CD4 SP), and CD8 SP thymocytes, whereas proportion of double positive (DP) had decreased (Fig. 2a, b ). These were attributed to the increased number of DN, CD4 SP, and CD8 SP thymocytes (Fig. 2c, d ). No obvious phenotypic differences were observed between WT and heterozygotes, between Δ E BAB males and Δ E BAB females, and among the three founder lines (Supplementary Fig. 3 ). Fig. 2 The Δ E BAB thymus accumulates high affinity TCR clones. a Flow cytometric analysis of CD4 versus CD8 thymocyte populations. Data are representative of seven independent experiments (Young; n = 7 WT and E BAB +/− –Δ E BAB littermate pairs, 7–17 weeks old) or five independent experiments (Aged; n = 5 WT & E BAB +/− –Δ E BAB littermate pairs, 30–36 weeks old). b – d Double negative (DN), double positive (DP), CD4 single positive (SP), and CD8 SP thymocyte proportions of young and aged mice ( b ), and cell numbers of young ( c ) and aged ( d ) mice. Data are pooled from seven independent experiments (Young; n = 7 WT and E BAB +/− –Δ E BAB littermate pairs, 7–17 weeks old) or five independent experiments (Aged; n = 5 WT and E BAB +/- –Δ E BAB littermate pairs, 30–36 weeks old). e Scatter plot (log 2 fold change versus –log 10 P value) of genes analyzed by RNA-seq ( n = 2 WT and E BAB +/− –Δ E BAB littermate pairs, 10–11 weeks old). Genes showing more than twofold changes with P < 0.05 (unpaired two-tailed Student’s t test) are highlighted. f Flow cytometric analysis of TCRβ versus CD69 thymocyte populations. Data are representative of five independent experiments (Young; n = 5 WT and E BAB +/− –Δ E BAB littermate pairs, 9–12 weeks old, Aged; n = 6 WT and E BAB +/− mice and n = 7 Δ E BAB mice from WT and E BAB +/− –Δ E BAB littermate pairs and trios, 30–36 weeks old). g Post-selection (TCRβ high CD69 high ) thymocyte proportion of young and aged mice. Data are pooled from five independent experiments (Young; n = 5 WT and E BAB +/− –Δ E BAB littermate pairs, 9–12 weeks old, Aged; n = 6 WT and E BAB +/− mice, n = 7 Δ E BAB mice, WT and E BAB +/− –Δ E BAB littermate pair or trio, 30–36 weeks old). h qPCR analysis for Nr4a1 in pre-selection (TCRβ low CD69 low ) and post-selection thymocytes of WT and Δ E BAB . Data are pooled from five independent experiments ( n = 5 sex-matched WT–Δ E BAB pairs, 10–18 weeks old, mean ± s.d.). Edges of the box are the 25th and 75th percentiles, and error bars extend to the maximum and minimum. Each symbol in ( b , c , d , g ) represents an individual mouse; small horizontal lines indicate the mean. n.s. not significant ( P ≥ 0.05); * P < 0.05, ** P < 0.01, *** P < 0.001 (unpaired two-tailed Student’s t test) Full size image To understand the nature of altered T cell homeostasis in the Δ E BAB thymus, we performed whole transcriptome analysis of Δ E BAB thymocytes (two littermate pairs) utilizing RNA-seq (Fig. 2e ). As shown in Fig. 2e , only a small number of genes showed statistically significant ( P < 0.05) more than twofold changes (see methods and Supplementary Data 2 for the detail). Yet, differentially expressed genes (DEGs) affected by Δ E BAB indicated that the Δ E BAB thymus accumulated high affinity TCR clones (Fig. 2e ): the Δ E BAB thymus exhibited a higher level of Nr4a1 expression when compared to the WT thymus. Nr4a1 is a faithful responder for TCR signal, and the expression level of Nr4a1 positively correlates with TCR signal strength [15] , [25] , [26] . Elevated expression of Nr4a1 is thus one of the hallmarks of high affinity TCR clones in the thymus. Arhgap20 and Tnfrsf9 , the top two most elevated genes in RNA-seq data in the Δ E BAB thymus (Fig. 2e ), are also known as being upregulated in TCR-activated T cells [26] , supporting the notion that high-affinity TCR clones accumulate in Δ E BAB mice. To obtain more evidence that the Δ E BAB thymus piles up high-affinity TCR clones, we stained thymocytes with anti-TCRβ and anti-CD69 antibodies (Fig. 2f, g ). We found that proportion of post-selection (TCRβ high CD69 high ) thymocytes was increased in the Δ E BAB thymus both in young and aged mice (Fig. 2f, g ). Moreover, as determined by cell-sorting followed by qPCR, Nr4a1 expression in post-selection thymocytes was much higher in Δ E BAB than in WT (Fig. 2h ). Thus, it was likely that high affinity TCR clones were accumulated in the Δ E BAB thymus. We also analyzed TCR + population in the DN subset: thymic precursors of TCRαβ + CD8αα + intestinal intraepithelial lymphocytes (IELs) [27] , [28] and TCR Vα14 + invariant natural killer T cells (iNKT cells) [29] , [30] . Our data demonstrated that Δ E BAB increased the number of IEL precursors (Supplementary Fig. 4a, b ), while iNKT population was much less affected by Δ E BAB (Supplementary Fig. 4c–e ). These changes may contribute to the increased number of DN thymocytes in Δ E BAB mice (Fig. 2c, d ). E BAB is required for eliminating high-affinity TCR clones Accumulation of high-affinity TCR clones in the Δ E BAB thymus led us to hypothesize that E BAB is required for negative selection and/or more general apoptosis processes. To test this hypothesis, we treated primary thymocytes with four apoptotic stimuli: dexamethasone (DEX) [7] , [8] , phorbol 12-myristate 13-acetate (PMA) [7] , [8] , ionomycin [7] , [8] (Supplementary Fig. 5 ), and anti-CD3 and anti-CD28 antibodies [6] , [25] (Fig. 3a ). Δ E BAB did not affect survival of DEX- or PMA-treated thymocytes (Supplementary Fig. 5a, b ) but partially rescued thymocytes from cell death caused by ionomycin or anti-CD3 and anti-CD28 antibodies (Fig. 3a and Supplementary Fig. 5c–e ). The rescue in ionomycin experiments was observed in a dose-dependent manner (Supplementary Fig. 5c–e ). PMA, ionomycin, and anti-CD3 and anti-CD28 antibodies are often used for artificially activating TCR stimulation and thus for mimicking negative selection ex vivo [6] , [7] , [8] , [25] . Thus, these results suggest that Δ E BAB thymocytes were defective in apoptosis following TCR signal activation, leading to a hypothesis that E BAB plays a role in depleting high-affinity TCR clones. Fig. 3 E BAB contributes to depletion of high affinity TCR clones in ex vivo TCR stimulation and the HY tg models. a Annexin V + Propidium Iodide (PI) − fraction of total thymocytes stimulated with anti-CD3 and anti-CD28 antibodies (10 µg/ml) for 9 h. The percentage in mock sample (i.e., background) is subtracted. Data are pooled from 11 independent experiments ( n = 3 WT–Δ E BAB littermate pairs, n = 3 sex-matched WT–Δ E BAB pairs, n = 1 WT– Bim −/− littermate pair, n = 1 sex-matched WT– Bim −/− pair, n = 3 sex-matched WT– Bim −/− –Δ E BAB trios, 5–20 weeks old). Edges of the box are the 25th and 75th percentiles, and error bars extend to the maximum and minimum. Outliers are defined as the data point that is located outside of q 3 + 1.5( q 3 − q 1 ) and q 1 − 1.5( q 3 − q 1 ), in which q 1 and q 3 are the 25th and 75th percentiles. b CD4 versus CD8 flow cytometric analysis of PI − HY-TCR + thymocytes from female and male HY tg mice. The number in the plot is representative percentage of each gate. c − d DP thymocyte proportion ( c ) and cell numbers ( d ) of PI − HY-TCR + thymocytes from female and male HY tg mice. e , f CD8 SP thymocyte proportion ( e ) and cell numbers ( f ) of PI − HY-TCR + thymocytes from female and male HY tg mice. Data are representative of ( b ), or pooled from ( c – f ), six independent experiments ( n = 1 Bim +/− ; HY + and Bim −/− ; HY + female mice, n = 5 Bim +/− ; HY + and Bim − /− ; HY + male mice, n = 3 E BAB +/− ; HY + and Δ E BAB ; HY + female mice, n = 5 E BAB +/− ; HY + and Δ E BAB ; HY + male mice, 6–8 weeks old). Each symbol in ( c – f ) represents an individual mouse; small horizontal lines indicate the means. n.s. not significant ( P ≥ 0.05); * P < 0.05, ** P < 0.01 (unpaired one-tailed Student’s t test or Mann–Whitney U test for Bim KO data, and unpaired two-tailed Student’s t test for Δ E BAB data) Full size image To assess the possibility that E BAB is required for deleting high affinity TCR clones in vivo, we took advantage of three TCR transgenic mouse models: HY transgenic (tg) [6] (Fig. 3b–f ), OT-II tg [6] , [31] , [32] (Fig. 4 ), and OT-I tg [33] , [34] , [35] (Supplementary Fig. 6 ). Fig. 4 E BAB is essential for depleting high affinity TCR clones in the OT-II tg model. a CD4 versus CD8 flow cytometric analysis of TCR Vβ5 + thymocytes from mice injected with OVA 257–264 or OVA 323–229 peptide intraperitoneally. The number in the plot is representative percentage of each gate. b CD4 SP thymocyte proportion of TCR Vβ5 + thymocytes from mice treated as in Fig. 4a. c TCRβ versus CD69 flow cytometric analysis of TCR Vβ5 + thymocytes from mice treated as in Fig. 4a. The number in the plot is representative percentage of the gate. d Post-selection (TCRβ high CD69 high ) thymocyte proportion of TCR Vβ5 + thymocytes from mice treated as in Fig. 4a. Data are representative of ( a , c ) or pooled from ( b , d ) 13 independent experiments ( n = 5 WT and E BAB +/− mice injected with OVA 257–264 peptide, n = 8 WT and E BAB +/− ; OT-II + mice injected with OVA 323–339 peptide, n = 6 Δ E BAB ; OT-II + mice injected with OVA 257–264 and OVA 323–339 peptide, n = 3 Bim +/− ; OT-II + and Bim −/− ; OT-II + mice injected with each peptide, 5–14 weeks old). Each symbol ( b , d ) represents an individual mouse; small horizontal lines indicate the mean. n.s. not significant ( P ≥ 0.05); ** P < 0.01, *** P < 0.001 (unpaired one-tailed Student’s t test for Bim KO data, unpaired two-tailed Student’s t test for Δ E BAB data) Full size image HY tg mice express αβTCRs that recognize a male-specific endogenous antigen called HY, which is presented by H-2D b class I MHC molecules [6] (Fig. 3b-f ). Δ E BAB ; HY tg mice were analyzed at 6–8 weeks old as described previously [6] by flow cytometry. As shown by the lower abundance of DP and CD8 SP in E BAB +/− ; HY tg male mice compared to female mice (Fig. 3b–f ), thymocytes expressing HY-TCR are negatively selected in a male-specific manner. Notably, Δ E BAB significantly rescued DP (both in proportion and number) and CD8 SP (in proportion) thymocytes in HY tg male mice (Fig. 3b–f ). OT-II tg thymocytes express Vα2/Vβ5 TCRs that primarily recognize chicken ovalbumin-derived peptide (ISQAVHAAHAEINEAGR, OVA 323–339 peptide) presented by I - A b class II MHC molecules [6] , [31] , [32] . Δ E BAB ; OT-II tg mice were generated by crossing and injected with OVA 323–339 peptide or the control peptide intraperitoneally. 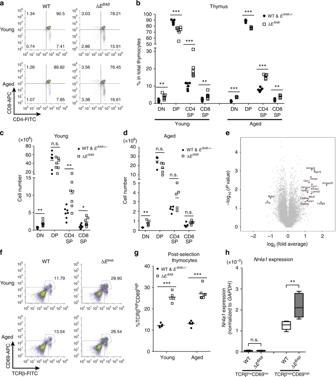Fig. 2 The ΔEBABthymus accumulates high affinity TCR clones.aFlow cytometric analysis of CD4 versus CD8 thymocyte populations. Data are representative of seven independent experiments (Young;n= 7 WT andEBAB+/−–ΔEBABlittermate pairs, 7–17 weeks old) or five independent experiments (Aged;n= 5 WT &EBAB+/−–ΔEBABlittermate pairs, 30–36 weeks old).b–dDouble negative (DN), double positive (DP), CD4 single positive (SP), and CD8 SP thymocyte proportions of young and aged mice (b), and cell numbers of young (c) and aged (d) mice. Data are pooled from seven independent experiments (Young;n= 7 WT andEBAB+/−–ΔEBABlittermate pairs, 7–17 weeks old) or five independent experiments (Aged;n=5 WT andEBAB+/-–ΔEBABlittermate pairs, 30–36 weeks old).eScatter plot (log2fold change versus –log10Pvalue) of genes analyzed by RNA-seq (n= 2 WT andEBAB+/−–ΔEBABlittermate pairs, 10–11 weeks old). Genes showing more than twofold changes withP< 0.05 (unpaired two-tailed Student’sttest) are highlighted.fFlow cytometric analysis of TCRβ versus CD69 thymocyte populations. Data are representative of five independent experiments (Young;n= 5 WT andEBAB+/−–ΔEBABlittermate pairs, 9–12 weeks old, Aged;n= 6 WT andEBAB+/−mice andn= 7 ΔEBABmice from WT andEBAB+/−–ΔEBABlittermate pairs and trios, 30–36 weeks old).gPost-selection (TCRβhighCD69high) thymocyte proportion of young and aged mice. Data are pooled from five independent experiments (Young;n= 5 WT andEBAB+/−–ΔEBABlittermate pairs, 9–12 weeks old, Aged;n= 6 WT andEBAB+/−mice,n= 7 ΔEBABmice, WT andEBAB+/−–ΔEBABlittermate pair or trio, 30–36 weeks old).hqPCR analysis forNr4a1in pre-selection (TCRβlowCD69low) and post-selection thymocytes of WT and ΔEBAB. Data are pooled from five independent experiments (n= 5 sex-matched WT–ΔEBABpairs, 10–18 weeks old, mean ± s.d.). Edges of the box are the 25th and 75th percentiles, and error bars extend to the maximum and minimum. Each symbol in (b,c,d,g) represents an individual mouse; small horizontal lines indicate the mean. n.s. not significant (P≥ 0.05); *P< 0.05, **P< 0.01, ***P< 0.001 (unpaired two-tailed Student’sttest) WT; OT-II tg or E BAB +/− ; OT-II tg mice were also used as a control. In response to injection with OVA 323–339 peptide, the CD4 SP proportion of control thymocytes was massively reduced (Fig. 4a, b ). Strikingly, E BAB KO rescued this reduction (Fig. 4a, b ). Staining thymocytes with anti-TCRβ and anti-CD69 antibodies revealed that Δ E BAB almost completely prevented the deletion of post-selection thymocytes caused by OVA 323–339 peptide injection (Fig. 4c, d ). Fetal thymic organ culture (FTOC) with the OT-I tg system allows us to investigate effects of antigens of interests on intrathymic T cell development [33] , [34] , [35] , [36] . OT-I tg thymocytes express Vα2/Vβ5 TCRs that bind chicken ovalbumin peptide residues 257–264 (SIINFEKL, OVA 257–264 peptide) in the context of H-2K b class I MHC molecules [34] . Of note, a series of OVA 257–264 variants with different TCR affinity can be used in the OT-I tg FTOC system [34] , [35] . We cultured fetal thymus (FT) of E BAB +/− ; OT-I tg and Δ E BAB ; OT-I tg in the presence of OVA 257–264 , Q4R7 (SIIQFERL), or gp33 (KAVYNFATC) [34] (Supplementary Fig. 6 ). The previous publications establish OVA 257–264 and Q4R7 as negative selectors (affinity to OT-I TCR: OVA 257–264 > Q4R7) [34] , [35] . gp33, which does not bind to OT-I TCRs, was used as a control. Δ E BAB compared to E BAB+/− significantly rescued DP thymocytes from Q4R7-dependent selection but not those from OVA 257–264 -dependent selection (Supplementary Fig. 6 ). Thus, Δ E BAB rescued OT-I TCR + thymocytes from negative selection in a TCR affinity-dependent manner. Taken the results from the three transgenic models together, we concluded that E BAB plays an important role in apoptosis of high-affinity TCR clones in thymic negative selection ex vivo and in vivo. E BAB is essential for TCR-dependent activation of Bim The above-described phenotypes observed in the Δ E BAB thymus, four ex vivo culture systems, and three transgenic models are strikingly similar to those observed in Bim KO mice as described in multiple publications [6] , [7] , [8] , [9] , [10] and as validated by ourselves (Figs. 2 – 4 and Supplementary Figs. 4 – 7 ). For example, the extent of increase for post-selection thymocytes caused by Δ E BAB was similar to that by Bim KO (Fig. 2g . versus Supplementary Fig. 7e ). Such similarity was also observed for the ex vivo TCR stimulation (Fig. 3a ), OT-II (Fig. 4 ), and OT-I (Supplementary Fig. 6 ) experiments, whereas Bim KO seemingly more efficiently rescued HY-TCR + thymocytes than E BAB KO did in the HY experiments (Fig. 3 : see discussion regarding interpretation on this data). Moreover, Δ E BAB did not affect DEX-induced cell death, which was in fact Bim -independent (Supplementary Fig. 5a ). Some of the thymocytes abnormalities are seen also in mice ectopically expressing Bim-antagonist Bcl2 (Bcl2 tg) in a T cell-specific manner, which leads to defective apoptosis in the thymus [25] , [37] , [38] . Although Δ E BAB had a minor impact on Bim expression in total thymocytes (Fig. 1e ), we next examined whether the deficient negative selection of Δ E BAB thymocytes is due to abnormal regulation of Bim . To this end, we again artificially activated TCR by treating thymocytes with anti-CD3 and anti-CD28 antibodies ex vivo, and then measured expression of Bim , Nr4a1 , Bub1 , and Bcl2 by qPCR (Fig. 5a–d ). Bim expression in Δ E BAB thymocytes treated with anti-CD3 and anti-CD28 antibodies was clearly lower than that in TCR-stimulated WT thymocytes (Fig. 5a ). Expression of Nr4a1 , a faithful responder for TCR signal, was comparable between WT and Δ E BAB (Fig. 5b ), suggesting that TCR signal was properly activated in Δ E BAB thymocytes. Consistent with the report that a dominant negative form of Bub1 is insufficient to cause T cell abnormalities [39] , Bub1 expression was not influenced by TCR stimulation and E BAB KO (Fig. 5c ). Bcl2 , a TCR-downstream anti-apoptotic gene, exhibited an expected response to TCR stimulation [40] , and this response was comparable between WT and Δ E BAB (Fig. 5d ). Thus, it was likely that E BAB primarily targets Bim following TCR signal. Fig. 5 E BAB regulates Bim expression upon TCR stimulation. a – d Gene expression changes for Bim ( a ), Nr4a1 ( b ), Bub1 ( c ), and Bcl2 ( d ) in total thymocytes stimulated for 3 h with anti-CD3 and anti-CD28 antibodies (10 µg/ml). e , f Gene expression level ( e ) and relative gene expression to WT ( f ) for Bim in pre-selection (TCRβ low CD69 low ) and post-selection (TCRβ high CD69 high ) thymocytes. g , h Gene expression level ( g ) and relative gene expression to WT ( h ) for Bub1 in pre-selection (TCRβ low CD69 low ) and post-selection (TCRβ high CD69 high ) thymocytes. Data are pooled from six independent experiments ( a – d ; n = 6 sex-matched WT–Δ E BAB pairs, 9–18 weeks old) or five independent experiments ( e – h ; n = 5 sex-matched WT–Δ E BAB pairs, 10–18 weeks old). Edges of the box are the 25th and 75th percentiles, and error bars extend to the maximum and minimum. Outliers are defined as the data point that is located outside of q 3 + 1.5( q 3 − q 1 ) and q 1 − 1.5( q 3 − q 1 ), in which q 1 and q 3 are the 25th and 75th percentiles. n.s. not significant ( P ≥ 0.05); * P < 0.05, ** P < 0.01, *** P < 0.001 (unpaired two-tailed Student’s t test) Full size image To assess the role of E BAB in TCR-dependent Bim activation in vivo, we sorted pre- and post-selection thymocytes and measured expression of Bim and Bub1 (Fig. 5e–h ). If E BAB regulates Bim in a TCR signal dependent manner, Bim expression should be affected by Δ E BAB at the post-selection stage while less affected at the pre-selection stage. As expected, expression of Bim in the post-selection (TCRβ high CD69 high ) thymocytes was markedly lower in Δ E BAB than in WT (Δ E BAB /WT = 0.31) (Fig. 5e, f ). Although Bim expression was moderately affected by E BAB KO in the pre-selection (TCRβ low CD69 low ) stage (Δ E BAB /WT = 0.64) (Fig. 5e, f ), expression ratio of Δ E BAB to WT in the post-selection stage was significantly lower than that in the pre-selection stage (Fig. 5f ). These results were validated at the protein level, demonstrating that protein expression of BimEL and BimL, two of major isoforms of Bim [41] , was compromised by Δ E BAB (Supplementary Fig. 9 ). Together, Δ E BAB affected Bim expression in a post-selection-biased manner, indicating an important role of E BAB in activating Bim upon TCR activation in vivo. Bub1 expression was not significantly altered between Δ E BAB and WT mice both in pre- and post-selection thymocytes (Fig. 5g, h ), again excluding Bub1 in explaining the T cell phenotypes we observed (Figs. 2 – 4 ). Collectively, our data demonstrated that E BAB KO disrupts transcriptional activation for Bim upon TCR stimulation, resulting in the rescue of high affinity TCR clones in the thymus (Figs. 2 – 5 ). We reasoned that Bim expression in total thymocytes looked only mildly affected by E BAB KO (Fig. 1e ) as only 10–30% of thymocytes is at the post-selection stage where transcriptional regulation of Bim is strongly affected by Δ E BAB . Furthermore, we investigated whether E BAB regulates Bim in cis or trans . To test this, we generated E BAB +/− ; Bim −/+ mice (Supplementary Fig. 10a ). If E BAB controls Bim in cis , a phenotype of E BAB +/− ; Bim −/+ thymocytes should be similar to Δ E BAB (Supplementary Fig. 10a ). If E BAB can regulate Bim in trans , E BAB +/− ; Bim −/+ mice should show no phenotype in the thymus (Supplementary Fig. 10a ). Staining with anti-CD4, anti-CD8, anti-TCRβ, and anti-CD69 antibodies revealed that E BAB +/ − ; Bim − /+ thymocytes exhibited Δ E BAB -like phenotypes (Supplementary Fig. 10b–f ). Given that Bim +/− exhibits almost no phenotype in DN, DP, CD4 SP, CD8 SP, and TCRβ high CD69 high thymocytes (Supplementary Fig. 10g ), these results validated that E BAB is a cis -regulatory element regulating Bim . E BAB is dispensable for T reg cells and peripheral T cells Expression levels of Nr4a transcription factors including Nr4a1 are markers not only for high affinity TCR clones, but also for thymic T reg cells that suppress autoreactive T cells in periphery [1] , [5] . Nr4a transcription factors cooperatively promote T reg differentiation through directly activating expression of Foxp3 , the master regulator for T reg identity [42] , [43] , [44] . Thus, it is thought that high-affinity TCR clones are a precursor of T reg cells [5] . Bim KO and Bcl2 tg mice accumulate both of high affinity TCR clones and T reg cells [6] , [7] , [8] , [14] , [15] , [25] , [37] , [38] (Supplementary Figs. 7d , e, 8c ). To examine whether accumulation of high-affinity TCR clones resulted in the increased number of T reg cells in Δ E BAB mice, we analyzed thymic and splenic T reg cells by staining with anti-Foxp3 antibody (Fig. 6a, b ). We found that the number of thymic and splenic T reg cells were comparable between WT and Δ E BAB (Fig. 6a, b ). Thus, although high-affinity TCR clones are accumulated in the Δ E BAB thymus (Fig. 2 ), E BAB does not affect homeostasis of T reg cells. These results indicate that Bim -dependent homeostasis of T reg cells in the thymus and spleen is independent on E BAB . Fig. 6 E BAB does not play a major role in maintaining homeostasis of regulatory T cells and peripheral T cells. a , b CD4 + Foxp3 + thymic ( a ) and splenic ( b ) T reg cell numbers of young and aged mice. Data are pooled from five independent experiments (Young; n = 5 WT and E BAB +/− –Δ E BAB littermate pairs, 9–12 weeks old, Aged; n = 5 WT E BAB +/− –Δ E BAB littermate pairs, 30–36 weeks old). c Flow cytometric analysis of CD4 versus CD8 T cell populations in the spleen. The number in the plot is representative percentage of each gate. Data are representative of five independent experiments (Young; n = 5 WT and E BAB +/− –Δ E BAB littermate pairs, 7–17 weeks old, Aged; n = 5 WT and E BAB +/− –Δ E BAB littermate pairs, 30–36 weeks old). d CD4 + and CD8 + splenic T cell numbers. Data are pooled from five independent experiments (Young; n = 5 WT and E BAB +/− –Δ E BAB littermate pairs, 7–17 weeks old, Aged; n = 5 WT and E BAB +/− –Δ E BAB littermate pairs, 30–36 weeks old). Each symbol in ( a , b , d ) represents an individual mouse; small horizontal lines indicate the mean. n.s. not significant ( P ≥ 0.05) (unpaired two-tailed Student’s t test) Full size image Bim KO and Bcl2 tg mice also accumulate peripheral T cells [6] , [7] , [8] , [12] , [13] , [25] , [37] , [38] (Supplementary Fig. 8a, b ). However, the number of splenic CD4 + and CD8 + T cell were not affected by Δ E BAB both in young and aged mice (Fig. 6c, d ). In addition, splenic B cells, whose homeostasis depends on Bim [8] , were unaffected by E BAB KO (Supplementary Fig. 11 ). These results indicated that homeostasis of peripheral T cells is properly maintained in Δ E BAB mice in contrast to Bim KO mice [6] , [7] , [8] , [12] , [13] (Supplementary Fig. 8a, b ). To gain an additional insight into a role of E BAB in peripheral T cell homeostasis, we performed Interleukin-2 (IL-2) deprivation experiments and activation-induced cell death (AICD) experiments in cultured activated CD4 + and CD8 + splenocytes (Fig. 7 ). Fig. 7 E BAB is dispensable for two apoptotic pathways in peripheral T cells. a , b Viability (% Annexin V − PI − ) of activated CD4 + ( a ) and CD8 + ( b ) splenic T cells after IL-2 withdrawal. Data are pooled from ten independent experiments ( a ; n = 5 sex-matched WT–Δ E BAB pairs and n = 5 sex-matched WT– Bim − /− –Δ E BAB trios, 5–26 weeks old, mean ± s.d.) or 11 independent experiments ( b ; n = 5 sex-matched WT–Δ E BAB pairs and n = 5 sex-matched WT– Bim −/− –Δ E BAB trios, 5–26 weeks old, mean ± s.d.). c , d Gene expression level for Bim in activated CD4 + ( c ) and CD8 + ( d ) splenic T cells cultured with or without IL-2 for 6 h. Data are pooled from five independent experiments ( n = 5 sex-matched WT– Bim − /− –Δ E BAB trios, 5–14 weeks old). e, f Expression of Bub1 in activated CD4 + ( e ) and CD8 + ( f ) splenic T cells cultured with or without IL-2 for 6 h. Data are pooled from five independent experiments ( n = 5 sex-matched WT– Bim −/− –Δ E BAB trios, 5–14 weeks old). g , h Apoptotic cell rate (%Annexin V + ) of activated CD4 + ( g ) and CD8 + ( h ) splenic T cells restimulated with anti-CD3 antibody (5 µg/ml) for 6 h. Data are pooled from five independent experiments ( n = 5 sex-matched WT– Bim −/− –Δ E BAB trios, 5–26 weeks old). Edges of the box are the 25th and 75th percentiles, and error bars extend to the maximum and minimum. Outliers are defined as the data point that is located outside of q 3 + 1.5( q 3 − q 1 ) and q 1 − 1.5( q 3 − q 1 ), in which q 1 and q 3 are the 25th and 75th percentiles ( c – h ). n.s. not significant ( P ≥ 0.05); * P < 0.05, ** P < 0.01, *** P < 0.001 (unpaired two-tailed Student’s t test) Full size image Bim -deficient peripheral T cells are resistant to the absence of IL-2 ex vivo [7] , [45] while WT and Δ E BAB splenic T cells needed IL-2 for their continuous survival in culture (Fig. 7a, b ). In accordance with this, E BAB was dispensable for upregulation of Bim following IL-2 withdrawal (Fig. 7c, d ). Expression of Bub1 was merely affected by IL-2 (Fig. 7e, f ). Hence, IL-2 deprivation-dependent T cell death in periphery requires Bim but not E BAB . AICD is known as a peripheral cell death cascade where repeatedly activated T cells undergo apoptosis [46] . In fact, reactivating peripheral T cells by anti-CD3 antibody treatment strongly induced cell death (Fig. 7g, h ). Using this system, we found that neither Bim nor E BAB was required for AICD ex vivo (Fig. 7g, h ). From these experiments, we concluded that at least two peripheral apoptotic pathways are intact in Δ E BAB mice, which can be one explanation for why the increase in thymic high-affinity TCR clones did not lead to accumulation of peripheral T cells. We additionally analyzed splenic activated T cell proportion by staining splenocytes with anti-CD44 and anti-CD62L antibodies to investigate autoimmune pathology (Fig. 8a–c ). In line with the fact that two peripheral apoptosis pathways are intact in Δ E BAB mice (Fig. 7 ), activated T cell (CD44 high CD62L low ) proportion was not increased in the Δ E BAB spleen even in aged mice (Fig. 8a–c and Supplementary Fig. 12a–e ). These data were in line with RNA-seq data from WT and Δ E BAB spleen (two littermate pairs), where only two candidate DEGs were identified (Supplementary Fig. 12f and Supplementary Data 3 ). In contrast, Bim -deficient mice accumulated activated CD8 + T cells in the spleen already at younger age (Supplementary Fig. 8d–f ). Fig. 8 Δ E BAB mice do not show any autoimmune phenotype. a Flow cytometric analysis of CD62L versus CD44 populations in CD4 + or CD8 + splenic T cell. The number in the plot is representative percentage of each gate. For CD4 + T cells, gates indicate activated (CD44 high CD62L low ) and naïve (CD44 low CD62L high ) populations. For CD8 + T cells, activated effector memory (CD44 high CD62L low ), activated central memory (CD44 high CD62L high ) and naïve (CD44 low CD62L high ) populations are gated. Data are representative of four independent experiments ( n = 5 for WT and E BAB +/− mice, n = 6 for Δ E BAB mice from WT & E BAB +/− –Δ E BAB littermate pairs and trios, 30–34 weeks old). b , c Activated CD4 + ( b ) and CD8 + ( c ) proportions of aged mice. Data are pooled from four independent experiments ( n = 5 for WT and E BAB +/− mice, n = 6 for Δ E BAB mice from WT and E BAB +/− –Δ E BAB littermate pairs and trios, 30–34 weeks old). d The mean (±s.e.m.) clinical scores at the days after EAE was induced in WT (control) ( n = 10) and Δ E BAB mice ( n = 8). The incidence of EAE: control 10/10, Δ E BAB 8/8. No data point showed statistically significant difference between WT and Δ E BAB (i.e., unpaired two-tailed Student’s t test P ≥ 0.05). e Representative pictures for Hematoxylin and Eosin staining for the lung, liver, kidney, and pancreas of two independent experiments ( n = 2 WT and E BAB +/− –Δ E BAB littermate pairs, 30–31 weeks old). The scale bars represent 100 μm. Each symbol in ( b , c ) represents an individual mouse; small horizontal lines indicate the mean. n.s. not significant ( P ≥ 0.05) (unpaired two-tailed Student’s t test) Full size image Furthermore, we assessed a role of E BAB in an in vivo autoimmune disease model, experimental autoimmune encephalomyelitis (EAE) [47] . As shown in Fig. 8d , clinical scores of Δ E BAB were comparable to those of WT: Δ E BAB mice neither exhibited severer nor ameliorated EAE phenotypes, suggesting that E BAB is dispensable for EAE. In contrast, we confirmed previous publication that Bim plays a role in EAE (Supplementary Fig. 13 ) [16] . Consistently, we did not find any histological sign for autoimmunity such as massive infiltration of leukocytes (i.e., inflammation) in several nonlymphoid organs in Δ E BAB mice (Fig. 8e ). Thus, Δ E BAB mice did not show any autoimmune phenotype, which was consistent with that E BAB was not essential for peripheral T cell homeostasis (Figs. 6 – 8 , Supplementary Fig. 8 , and Supplementary Figs. 12 and 13 ). These results highlighted an extraordinary specialized role of E BAB in thymic negative selection (Fig. 9 ). Fig. 9 Graphical summary. E BAB plays a role in inducing TCR signal-dependent apoptosis to eliminate high affinity TCR clones in the thymus while dispensable for Bim -dependent peripheral T cell tolerance Full size image It is thought that TCR signal activates Bim to promote apoptosis in thymic negative selection process [1] , [2] , [3] . However, it has been unclear how TCR signal strength is linked to the Bim expression level. Even whether activation of Bim expression is critical for negative selection has been unanswered due to lack of a mutant specifically deficient for TCR-dependent Bim expression [17] . Here, by means of CRISPR–Cas9-mediated KO approach in mice, we generated a mutant that lacks a cis -regulatory enhancer for Bim , E BAB (Figs. 1 – 5 and Supplementary Fig. 10 ). E BAB is T cell-specific and evolutionarily conserved (Fig. 1a, b and Supplementary Fig. 1 ), and Δ E BAB mice were unable to efficiently eliminate high affinity TCR clones (Figs. 2 – 4 and Supplementary Fig. 6 ). This defect appeared to be attributed to insufficient activation of Bim during TCR activation (Fig. 5 and Supplementary Fig. 9 ). Thus, we propose that E BAB links TCR signal and Bim expression, contributing to depletion of high affinity TCR clones in the thymus and thus to central T cell tolerance (Fig. 9 ). Bim KO affects homeostasis of nearly all of T cell types [6] , [7] , [8] , [9] , [10] , [11] , [12] , [13] , [14] , [15] , [16] , [17] , [18] (Supplementary Fig. 4 and Supplementary Figs. 7 and 8 ). Comparing T cell phenotypes between Bim KO and Δ E BAB mice provides insights into the extent of contribution of E BAB -dependent Bim regulation on phenotypes of interests. Among the phenotypes observed in the Δ E BAB thymus, accumulation of post-selection thymocytes in the Δ E BAB thymus was as severe as that in the Bim KO thymus (Fig. 2f, g and Supplementary Fig. 7d, e ). Moreover, both of Δ E BAB and Bim KO rescued thymocytes from negative selection in the ex vivo TCR stimulation model and three transgenic systems (Figs. 3 and 4 and Supplementary Fig. 6 ). The degrees of rescues by E BAB KO and Bim KO were similar in the ex vivo TCR stimulation, OT-I, and OT-II experiments (Figs. 3 and 4 and Supplementary Fig. 6 ). In contrast, in the HY experiments, it appeared that Bim KO better rescued HY-TCR + thymocytes than E BAB KO. When interpreting these results, it should be noted that readouts used (e.g., proportion of cell types of interests) do not always specifically reflect negative selection. In particular, Bim KO is able to rescue apoptosis induced by various stimuli [18] , even death of control-treated cells (Supplementary Fig. 5 ). Thus, increased survival seen in Bim KO potentially reflects both negative selection-dependent and -independent events such as post-selection lifetime. Importantly, our analyses showed that function of E BAB appears to be specific for TCR signal-dependent Bim expression in the thymus. Hence, we assume that the more efficient rescue observed in Bim KO in the HY experiments may be attributed to pleiotropic effects of Bim KO on negative selection-independent phenomena in the thymus. Alternatively, the observations in the HY experiments imply that there may be another enhancer controlling TCR-dependent expression of Bim . Collectively, we suggest that a role for Bim in eliminating high affinity TCR clones in the thymus requires E BAB . These results establish E BAB -mediated transcriptional regulation for Bim as a contributor for Bim -dependent thymic negative selection. Bim KO and Bcl2 tg mice accumulate T reg cells, a basis for the current model that T reg cells are differentiated from high-affinity TCR clones in the thymus [1] , [5] , [15] , [25] (Supplementary 8c ). Intriguingly, in the Δ E BAB thymus, the number of T reg cells was comparable with that in the littermate controls even though high affinity TCR clones were increased (Fig. 2f, g and Fig. 6a, b ). This indicates that the residual amount of Bim in the Δ E BAB thymus is sufficient for maintaining T reg homeostasis. It is also plausible that a non-cell autonomous mechanism may be dominant for T reg homeostasis in the thymus. Supporting this, a previous study shows that Foxp3 overexpression induces Bim phosphorylation and enhances apoptosis in newly arising thymic T reg cells [48] . In addition, T reg homeostasis is controlled by availability of pro-survival cytokines such as IL-2 derived from the surrounding environment [48] , [49] . These altogether indicate that T reg apoptosis is precisely tuned by multiple mechanisms independent from E BAB , and demonstrate that the role of E BAB is specific for thymic negative selection (Fig. 9 ). Alternatively, the increased proportion of IEL precursors both in Bim −/− and Δ E BAB mice (Supplementary Fig. 4a, b ) suggests that E BAB controls fate determination of survived high-affinity TCR clones: Δ E BAB may bias fate of thymocytes escaped from negative selection toward IEL rather than T reg cells. Bim KO and Bcl2 tg mice show abnormalities not only in thymic negative selection, but also in peripheral T cell homeostasis [6] , [7] , [8] , [11] , [12] , [13] , [25] , [37] , [38] (Supplementary Fig. 8a, b and Supplementary Fig. 12 ). In contrast, peripheral T cells did not accumulate in the Δ E BAB spleen (Fig. 6c, d ). Consistent with this, Δ E BAB affects neither peripheral T cell activation nor experimental autoimmunity (Fig. 8 and Supplementary Fig. 12 ). This suggests that high-affinity TCR clones were peripherally depleted in Δ E BAB mice. One possible explanation for this observation is that peripherally activated T cells properly undergo IL-2 withdrawal-dependent apoptosis, a process that requires Bim but not E BAB (Fig. 7a, b ). This idea is further supported by that Bim was properly upregulated upon IL-2 withdrawal in activated T cells even in the absence of E BAB (Fig. 7c, d ). Additional peripheral T cell-specific enhancer(s) for Bim , or completely different mechanisms such as post-translational modifications, may also ensure Bim -mediated maintenance for peripheral T cell homeostasis. A different apoptosis pathway such as the Fas pathway could also be a major contributor in eliminating peripheral autoreactive T cells [1] , [46] , [50] , [51] . 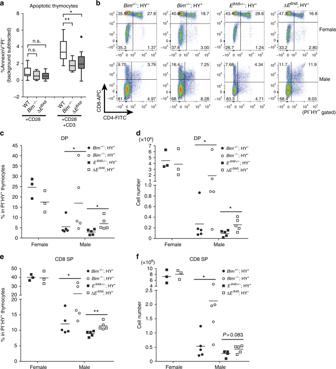Fig. 3 EBABcontributes to depletion of high affinity TCR clones in ex vivo TCR stimulation and the HY tg models.aAnnexin V+Propidium Iodide (PI)−fraction of total thymocytes stimulated with anti-CD3 and anti-CD28 antibodies (10 µg/ml) for 9 h. The percentage in mock sample (i.e., background) is subtracted. Data are pooled from 11 independent experiments (n= 3 WT–ΔEBABlittermate pairs,n= 3 sex-matched WT–ΔEBABpairs,n= 1 WT–Bim−/−littermate pair,n= 1 sex-matched WT–Bim−/−pair,n= 3 sex-matched WT–Bim−/−–ΔEBABtrios, 5–20 weeks old). Edges of the box are the 25th and 75th percentiles, and error bars extend to the maximum and minimum. Outliers are defined as the data point that is located outside ofq3+ 1.5(q3−q1) andq1− 1.5(q3−q1), in whichq1andq3are the 25th and 75th percentiles.bCD4 versus CD8 flow cytometric analysis of PI−HY-TCR+thymocytes from female and male HY tg mice. The number in the plot is representative percentage of each gate.c−dDP thymocyte proportion (c) and cell numbers (d) of PI−HY-TCR+thymocytes from female and male HY tg mice.e,fCD8 SP thymocyte proportion (e) and cell numbers (f) of PI−HY-TCR+thymocytes from female and male HY tg mice. Data are representative of (b), or pooled from (c–f), six independent experiments (n= 1Bim+/−; HY+andBim−/−; HY+female mice,n= 5Bim+/−; HY+andBim−/−; HY+male mice,n= 3EBAB+/−; HY+and ΔEBAB; HY+female mice,n= 5EBAB+/−; HY+and ΔEBAB; HY+male mice, 6–8 weeks old). Each symbol in (c–f) represents an individual mouse; small horizontal lines indicate the means. n.s. not significant (P≥ 0.05); *P< 0.05, **P< 0.01 (unpaired one-tailed Student’sttest or Mann–WhitneyUtest forBimKO data, and unpaired two-tailed Student’sttest for ΔEBABdata) The Fas pathway is known to be required for AICD, which we found requires neither Bim nor E BAB (Fig. 7g, h ). These results are consistent with that deletion of E BAB had a very minor impact on genome-wide gene expression in peripheral T cells (Supplementary Fig. 12f ). Collectively, our findings emphasize that the role of E BAB is dedicated to thymic negative selection (Fig. 9 ). A physiological contribution of a gene in a certain biological phenomenon depends on quantity of functional gene products that exist in that context. Regarding classical protein-coding genes, concentration of functional gene products-(modified) proteins is affected by transcriptional regulation, mRNA stability, translational efficacy, post-translational modifications, and protein stability, which are interconnected with each other. Each of these mechanisms profoundly contributes to determine the steady-state concentration of gene products, depending on genes and biological contexts. However, it has been technically difficult to dissect the relative importance of each mechanism for a gene to exert its physiological role(s) in a certain biological situation. Our study is unique in that we disrupted the single gene expression program by targeting the specific cis -element. This enabled us to reveal the degrees of contribution of Bim and E BAB in thymic negative selection measured by different readouts, which represent cutting-edge molecular dissection of the cis -regulatory control for thymic negative selection in vivo. Although we do not exclude a possibility that downstream mechanisms such as Bim phosphorylation might be also important, we provide the evidence that the enhancer-driven gene expression regulation of Bim is an important upstream mechanism in thymic negative selection. In addition, the present work provides an example for using enhancer KO approach, instead of conventional genetic-manipulation of protein-coding genes, to address important biological questions. Mice All animal protocols were approved by the Animal Care and Use committee of Advanced Telecommunications Research Institute International (permission numbers: AN20140002, AN20150002, AN20160002, AN20170002, and AN20180002) and Kyoto university (permission numbers: K-16-12-11 and L-18-1). For generating Δ E BAB mice, four gRNAs were individually cloned into the pX330 vector (#42230, Addgene, MA, USA) that harbors a Cas9 transgene. Briefly, two pairs of oligos (Supplementary Data 1 ) were annealed at 95 °C followed by natural cooling to 25 °C, and ligated with BbsI (New England Biolabs, MA, USA)-digested pX330 by using Ligation high (TOYOBO, Osaka, Japan). The obtained plasmids were sequence-validated (FASMAC, Kanagawa, Japan). The four gRNAs were together injected into fertilized eggs of C57BL/6N mice at the concentration of 2.5 μg/μl each (Transgenic, Fukuoka, Japan), generating the three different founders #44, #47, and #50. These founders were crossed with WT to obtain F1. Deleted regions were validated by sequencing analyses (FASMAC) against DNA from F0 and F1. The obtained F1 offspring were then crossed to generate Δ E BAB mice. Bim −/− (B6.129S1- Bcl2l11 tm1.1Ast /J) and OT-II tg (B6.Cg-Tg(TcrαTcrβ)425Cbn/J) mice were purchased from The Jackson Laboratory (ME, USA). OT-II tg, OT-I tg and HY tg mice were crossed with Δ E BAB and Bim −/ − mice for negative selection assays. In all mice experiments, KO and the littermate control (WT or heterozygote), thus in total two to three mice were sacrificed and analyzed side-by-side on the same day to be considered as a littermate pair or trio. All experiments were performed without randomization. Blinding was performed in the injection process of OT-II negative selection assay. In other experiments, blinding was not done. DNA isolation and genomic PCR Genomic DNAs were prepared by using MightyAMP DNA polymerase kit (TaKaRa, Shiga, Japan) according to the manufacturer’s instruction. Genomic PCR experiments were performed using MightyAMP DNA polymerase or KOD FX-neo (TOYOBO) and the primers listed in Supplementary Data 1 . Epigeome analysis Epigenome analyses were performed with the UCSC genome browser ( https://genome.ucsc.edu/ ). For analyzing epigenome from peripheral naïve T cells, ChIP-seq data retrieved (accession numbers: GSE67443 and GSE60005) were mapped to the mm9 of mouse genome by using Bowtie2 [52] . The obtained sam format files were converted into bam format files by using samtools [53] that were then subjected to peak calling with MACS [54] . Wig format files were then uploaded into the UCSC genome browser to be visualized. RNA isolation, cDNA synthesis, and qPCR For nonlymphoid organs, total RNAs were prepared by using Trizol reagent (Thermo Fisher Scientific, MA, USA). The obtained supernatants containing total RNAs were further purified with RNeasy mini kit (Qiagen, Venlo, Netherlands) according to the manufacturer’s instruction. Total RNAs from lymphocyte samples were prepared by RNeasy mini kit with the equipped lysis buffer. 0.1–2 μg of total RNAs were then reverse transcribed with SuperScript III first-strand synthesis system (Thermo Fisher Scientific) according to the manufacturer’s instruction. The obtained cDNAs were 5- or tenfold-diluted and subjected into qPCR experiments by using LightCycler480 Instrument II system and SYBR Green Master Mix (Roche, Basel, Switzerland). The obtained data were analyzed using the delta-Ct method. Antibodies Anti-CD4 antibody (Clone: GK1.5 (FITC), SONY, Tokyo, Japan), anti-CD8a antibody (Clone: 53-6.7 (APC), SONY), anti-CD8b antibody (eBioH35-17.2 (PE), Invitrogen, CA, USA), anti-TCRβ antibody (Clone: H57-597 (FITC), SONY), anti-TCRβ antibody (Clone: H57-597 (APC/Cy7), BioLegend, CA, USA), anti-CD69 antibody (Clone: H1.2F3 (APC), BioLegend), anti-CD5 antibody (Clone: 53-7.3 (APC), BioLegend), anti-CD44 antibody (Clone: IM7 (Alexa Fluor 700), BioLegend), anti-CD62L antibody (Clone: MEL-14 (PE), BioLegend), anti-TCR Vβ5.1, 5.2 antibody (Clone: MR9-4 (PE), BioLegend), anti-TCR HY antibody (Clone: T3.70 (PE), eBioscience, CA, USA), anti-B220 antibody (Clone: RA3-6B2 (FITC), SONY), LEAF-purified anti-CD3ε antibody (Clone: 145-2C11, BioLegend), LEAF-purified anti-CD28 antibody (Clone: 37.51, BioLegend), Biotin anti-TCRβ antibody (Clone: H57-597, BioLegend) and Biotin anti-CD69 antibody (Clone: H1.2F3, BioLegend) were used in this study. Flow cytometry The thymus and spleen were harvested to obtain single lymphocytes suspension. For splenocytes, red blood cells (RBCs) were lysed with RBC lysis buffer (0.015 M NH 4 Cl, 0.1 mM KHCO 3 , 0.01 mM Na 2 EDTA). Live cell numbers were counted by using Countess system (Thermo Fisher Scientific). 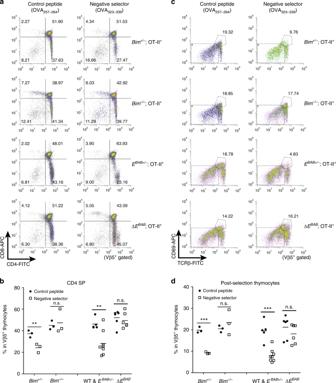Fig. 4 EBABis essential for depleting high affinity TCR clones in the OT-II tg model.aCD4 versus CD8 flow cytometric analysis of TCR Vβ5+thymocytes from mice injected with OVA257–264or OVA323–229peptide intraperitoneally. The number in the plot is representative percentage of each gate.bCD4 SP thymocyte proportion of TCR Vβ5+thymocytes from mice treated as in Fig. 4a.cTCRβ versus CD69 flow cytometric analysis of TCR Vβ5+thymocytes from mice treated as in Fig. 4a. The number in the plot is representative percentage of the gate.dPost-selection (TCRβhighCD69high) thymocyte proportion of TCR Vβ5+thymocytes from mice treated as in Fig. 4a. Data are representative of (a,c) or pooled from (b,d) 13 independent experiments (n= 5 WT andEBAB+/−mice injected with OVA257–264peptide,n= 8 WT andEBAB+/−; OT-II+mice injected with OVA323–339peptide,n= 6 ΔEBAB; OT-II+mice injected with OVA257–264and OVA323–339peptide,n= 3Bim+/−; OT-II+andBim−/−; OT-II+mice injected with each peptide, 5–14 weeks old). Each symbol (b,d) represents an individual mouse; small horizontal lines indicate the mean. n.s. not significant (P≥ 0.05); **P< 0.01, ***P< 0.001 (unpaired one-tailed Student’sttest forBimKO data, unpaired two-tailed Student’sttest for ΔEBABdata) The obtained samples (1 × 10 6 cells) were then stained with anti-CD4 antibody (1:200), anti-CD8a antibody (1:100), anti-CD8b antibody (1:200), anti-TCRβ antibody (1:200 (FITC), 1:100 (APC/Cy7)), anti-CD69 antibody (1:100), anti-CD5 antibody (1:100), anti-CD44 antibody (1:200), anti-CD62L antibody (1:100), anti-TCR Vβ5.1, 5.2 antibody (1:100), anti-TCR HY antibody (1:200) or anti-B220 antibody (1:100) in 100 μl of FCM buffer (10% fetal bovine serum (FBS) in phosphate-buffered saline (PBS)) for >30 min at 4 °C in the dark. For IEL precursors and iNKT measurement, 1 × 10 6 thymocytes were stained with α-GalCer-loaded CD1d tetramer (TS-MCD-1 (PE), MBL, Aichi, Japan) in 50 μl of FCM buffer for >30 min at 4 °C in the dark, and then stained with additional antibodies (see Supplementary Fig. 4 for the details). To analyze T reg cells, the obtained single cell suspension (3–5 × 10 6 cells) was stained using Foxp3 staining kit (Clone: FJK-16s, eBioscience, CA, USA), essentially according to the manufacturer’s instruction. Cell fixation was performed for 10 min. Samples were analyzed on EC800 (SONY) and FACS CantoII (BD Bioscience, NJ, USA). Gating strategies are shown in Supplementary Fig. 14 . RNA-seq and bioinformatic analysis Total RNAs were extracted from the thymus and spleen as described in the RNA isolation section. RNA-seq libraries were generated using the SureSelect Strand-Specific RNA Library Prep for Illumina (Agilent) according to the manufacturer’s instructions. Sequencing experiments were performed with Hiseq2500 (Illumina; Single End 36 bp). The obtained reads were mapped to the mouse genome mm9 using Illumina Eland with the default parameter setting. Uniquely aligned reads were retrieved allowing up to 2 bp mismatches, and the number of exon-mapped overlapping reads were counted. The obtained gene list with reads per million per a kilobase (RPKM) scores were shown in Supplementary Datas 2 and 3 . To identify DEGs, we first focused on the well-annotated protein-coding genes. RPKM scores from two replicates were averaged, and the ratio Δ E BAB /WT were calculated. In this calculation, 1 was added to all averaged RPKM scores to ignore scores below “1”, and to make analyses more stringent. The obtained ratios were used to sort genes to find candidate DEGs, followed by statistical analyses (unpaired two-tailed Student’s t -test) and qPCR validation. Cell sorting To purify pre- and post-selection thymocytes, single cell suspension (1–2 × 10 7 cells) was stained with anti-TCRβ antibody (1:100 or 1:200) and anti-CD69 antibody (1:100 or 1:200) in 100 μl of FCM buffer for >30 min at 4 °C in the dark. The stained cells were then tenfold diluted and sorted using SH800 cell sorter system (SONY). Ex vivo thymocytes cell death assay Totally, 1 × 10 5 total thymocytes were cultured with DEX (10 nM), PMA (2 ng/ml) or ionomycin (1 μg/ml or 0.1 μg/ml) in 200 μl of RPMI1640 media (10% FBS, 1% penicillin streptomycin, 50 μM 2-mercaptoethanol, 1 × nonessential amino acids (nacalai tesque, Kyoto, Japan) and 1 × sodium pyruvate (nacalai tesque)) in a 96-well flat bottom plate. DMSO- or EtOH-treated cells served as controls. Viability was measured by Annexin V FLUOS staining kit (Roche) at days 0–2. Ex vivo TCR stimulation Ex vivo TCR stimulation experiments were performed essentially as described previously [7] , [25] . Briefly, 12-well plates were coated with LEAF-purified anti-CD3ε and anti-CD28 antibodies (0 or 10 μg/ml in 500 μl of PBS, BioLegend) for 2 h at 37 °C. After 3 times-wash with 0.5 ml of PBS, 1 × 10 6 cells of total thymocytes were cultured in 2 ml of DMEM media (10% FBS, 1% penicillin streptomycin, 2 mM l -glutamine, 50 μM 2-mercaptoethanol, 10 mM HEPES (pH 7.4), 1 × nonessential amino acids (nacalai tesque) and 1 × sodium pyruvate (nacalai tesque)) for 3 h (for qPCR experiments) or 9 h (for Annexin V and PI staining using Annexin V FLUOS staining kit (Roche)). Peptides OVA 323–339 peptide (ISQAVHAAHAEINEAGR, BEX, Tokyo, Japan), OVA 257–264 peptide (SIINFEKL, BEX), gp33 (KAVYNFATC, BEX), and Q4R7 (SIIQFERL, BEX) were certified as >98% pure by HPLC. Peptides were dissolved in dimethyl sulfoxide (DMSO) at concentration of 100 mg/ml and stored at −80 °C. The peptide/DMSO solutions were diluted in PBS just before the experiment. OT-II negative selection assay OT-II negative selection assay was performed as described previously [6] . Briefly, WT; OT-II + , E BAB +/− ; OT-II + and Δ E BAB ; OT-II + mice were injected intraperitoneally with 1 mg OVA 323–339 peptide or OVA 257–264 peptide as a control resuspended in 500 μl of PBS. Thymocytes were harvested after 72 h for analysis. 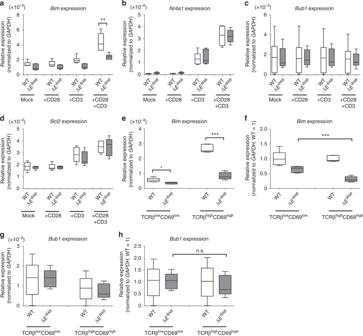Fig. 5 EBABregulatesBimexpression upon TCR stimulation.a–dGene expression changes forBim(a),Nr4a1(b),Bub1(c), andBcl2(d) in total thymocytes stimulated for 3 h with anti-CD3 and anti-CD28 antibodies (10 µg/ml).e,fGene expression level (e) and relative gene expression to WT (f) forBimin pre-selection (TCRβlowCD69low) and post-selection (TCRβhighCD69high) thymocytes.g,hGene expression level (g) and relative gene expression to WT (h) forBub1in pre-selection (TCRβlowCD69low) and post-selection (TCRβhighCD69high) thymocytes. Data are pooled from six independent experiments (a–d;n= 6 sex-matched WT–ΔEBABpairs, 9–18 weeks old) or five independent experiments (e–h;n= 5 sex-matched WT–ΔEBABpairs, 10–18 weeks old). Edges of the box are the 25th and 75th percentiles, and error bars extend to the maximum and minimum. Outliers are defined as the data point that is located outside ofq3+ 1.5(q3−q1) andq1− 1.5(q3−q1), in whichq1andq3are the 25th and 75th percentiles. n.s. not significant (P≥ 0.05); *P< 0.05, **P< 0.01, ***P< 0.001 (unpaired two-tailed Student’sttest) OT-I tg fetal thymic organ culture FTOC was performed as described previously [33] , [34] , [35] . Briefly, fetal thymic lobes were excised at embryonic day 15 (E15) and cultured on Whatman Nuclepore Track-Etched Membrane (WHA110409, GE Healthcare, Little Chalfont, England) floated on RPMI1640 media (10% FBS, 1% penicillin streptomycin, 50 μM 2-mercaptoethanol, 1 × nonessential amino acids (nacalai tesque, Kyoto, Japan) and 1 × sodium pyruvate (nacalai tesque)) in the presence of 2 μM OVA 257–264 , 2 μM Q4R7, or 20 μM gp33. On day 4, thymocytes were analyzed by flow cytometry. Immunoblotting assay CD69 + and CD69 − T cells were enriched from thymocytes using biotinylated anti-CD69 antibody (BioLegend) and MojoSort Streptavidin Nanobeads (BioLegend). CD69 - T cells were further purified by depleting TCRβ + cells using biotinylated anti-TCRβ antibody (BioLegend) and MojoSort Streptavidin Nanobeads (BioLegend). Expression of Bim and ACTB proteins in each subset was detected with anti-Bim antibody (1:1000, #2819, Cell Signaling, MA, USA) and anti-ACTB antibody (1:10,000, NB600-532, Novus Biologicals, CO, USA). As the secondary antibody, anti-rabbit IgG (1:15,000, 711-035-152, Jackson ImmumoResearch, PA, USA) was used. Signals were visualized with ECL plus Western Blotting Detection Reagents (GE Healthcare) and analyzed by the CCD digital imaging system LAS-4000 Luminescent Image Analyzer (GE Healthcare). Whole proteins were stained with SYPRO Ruby Protein Gel Stain (S12000, Thermo Fisher Scientific) and detected by the CCD digital imaging system LAS-4000 Luminescent Image Analyzer (GE Healthcare). Uncropped scans are available in the Source data file. Cytokine withdrawal assay CD4 + or CD8 + T cells were isolated from splenocytes using MojoSort Mouse CD4 or CD8 T Cell Isolation Kit (BioLegend), respectively according to the manufacturer’s instruction. T cells were activated by culturing cells in RPMI1640 media (10% FBS, 1% penicillin streptomycin, 50 μM 2-mercaptoethanol, 1 × nonessential amino acids (nacalai tesque) and 1 × sodium pyruvate (nacalai tesque)) plus IL-2 (100 U/ml, Wako, Osaka, Japan) in 96 well flat bottom plate coated with LEAF-purified anti-CD3ε and anti-CD28 antibodies (5 μg/ml in 50 μl of PBS, BioLegend) for 48 hr. 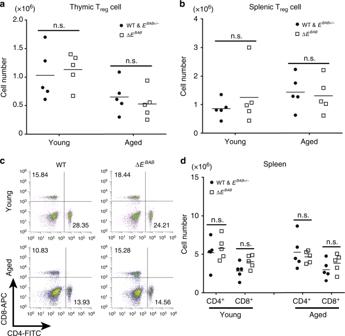Fig. 6 EBABdoes not play a major role in maintaining homeostasis of regulatory T cells and peripheral T cells.a,bCD4+Foxp3+thymic (a) and splenic (b) Tregcell numbers of young and aged mice. Data are pooled from five independent experiments (Young;n= 5 WT andEBAB+/−–ΔEBABlittermate pairs, 9–12 weeks old, Aged;n= 5 WTEBAB+/−–ΔEBABlittermate pairs, 30–36 weeks old).cFlow cytometric analysis of CD4 versus CD8 T cell populations in the spleen. The number in the plot is representative percentage of each gate. Data are representative of five independent experiments (Young;n= 5 WT andEBAB+/−–ΔEBABlittermate pairs, 7–17 weeks old, Aged;n=5 WT andEBAB+/−–ΔEBABlittermate pairs, 30–36 weeks old).dCD4+and CD8+splenic T cell numbers. Data are pooled from five independent experiments (Young;n= 5 WT andEBAB+/−–ΔEBABlittermate pairs, 7–17 weeks old, Aged;n=5 WT andEBAB+/−–ΔEBABlittermate pairs, 30–36 weeks old). Each symbol in (a,b,d) represents an individual mouse; small horizontal lines indicate the mean. n.s. not significant (P≥ 0.05) (unpaired two-tailed Student’sttest) Activated T cells were then cultured for 1 day with RPMI1640 plus IL-2 (100 U/ml, Wako) in normal 96-well plate. After that, IL-2 was removed from the media and viability of CD4 + and CD8 + T cells was measured using Annexin V FLUOS staining kit (Roche) on days 1–3 after IL-2 withdrawal. Activation induced cell death assay Isolation and activation of CD4 + or CD8 + T cells were performed as described in the “cytokine withdrawal assay” section. After activation and 1-day culture in the presence of IL-2, T cells were further incubated in RPMI1640 media (10% FBS, 1% penicillin streptomycin, 50 μM 2-mercaptoethanol, 1 × nonessential amino acids (nacalai tesque) and 1 × sodium pyruvate (nacalai tesque)) without IL-2 in a 96-well flat bottom plate coated with LEAF-purified anti-CD3ε (5 μg/ml in 50 μl of PBS, BioLegend) for 6 h. Cell viability was determined using Annexin V FLUOS staining kit (Roche). 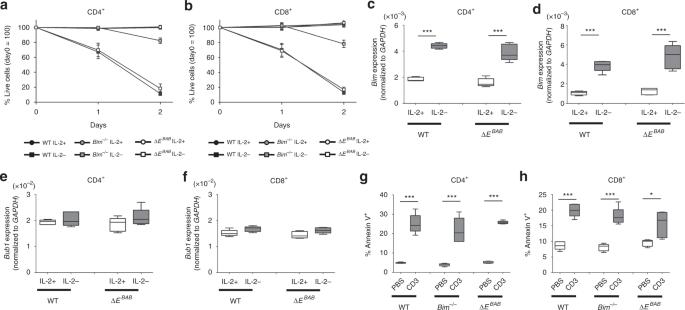Fig. 7 EBABis dispensable for two apoptotic pathways in peripheral T cells.a,bViability (% Annexin V−PI−) of activated CD4+(a) and CD8+(b) splenic T cells after IL-2 withdrawal. Data are pooled from ten independent experiments (a;n= 5 sex-matched WT–ΔEBABpairs andn= 5 sex-matched WT–Bim−/−–ΔEBABtrios, 5–26 weeks old, mean ± s.d.) or 11 independent experiments (b;n= 5 sex-matched WT–ΔEBABpairs andn= 5 sex-matched WT–Bim−/−–ΔEBABtrios, 5–26 weeks old, mean ± s.d.).c,dGene expression level forBimin activated CD4+(c) and CD8+(d) splenic T cells cultured with or without IL-2 for 6 h. Data are pooled from five independent experiments (n= 5 sex-matched WT–Bim−/−–ΔEBABtrios, 5–14 weeks old).e,fExpression ofBub1in activated CD4+(e) and CD8+(f) splenic T cells cultured with or without IL-2 for 6 h. Data are pooled from five independent experiments (n= 5 sex-matched WT–Bim−/−–ΔEBABtrios, 5–14 weeks old).g,hApoptotic cell rate (%Annexin V+) of activated CD4+(g) and CD8+(h) splenic T cells restimulated with anti-CD3 antibody (5 µg/ml) for 6 h. Data are pooled from five independent experiments (n= 5 sex-matched WT–Bim−/−–ΔEBABtrios, 5–26 weeks old). Edges of the box are the 25th and 75th percentiles, and error bars extend to the maximum and minimum. Outliers are defined as the data point that is located outside ofq3+ 1.5(q3 −q1) andq1− 1.5(q3−q1), in whichq1andq3are the 25th and 75th percentiles (c–h). n.s. not significant (P≥ 0.05); *P< 0.05, **P< 0.01, ***P< 0.001 (unpaired two-tailed Student’sttest) Histochemistry Mouse tissues were fixed in 10% neutral buffered formalin. Samples were then processed into 6 micron sections, mounted, and Hematoxylin and eosin (H&E)-stained (Genostaff, Tokyo, Japan). The prepared samples were observed with Nikon Ni-E microscope (Nikon, Tokyo, Japan). Experimental autoimmune encephalomyelitis Experimental autoimmune encephalomyelitis (EAE) experiments were performed essentially as described previously [47] . Briefly, mice (WT, Δ E BAB , and Bim −/ − ) were subjected to subcutaneous injection at two different sites with an emulsion of complete Freund’s adjuvant (CFA; 250 μg heat-killed Mycobacterium tuberculosis H37Ra (Difco) dissolved in 50 μl incomplete Freund’s adjuvant (Sigma)) and 250 μg myelin oligodendrocyte glycoprotein (MOG) peptides (amino acids 35–55) in 50 μl PBS. 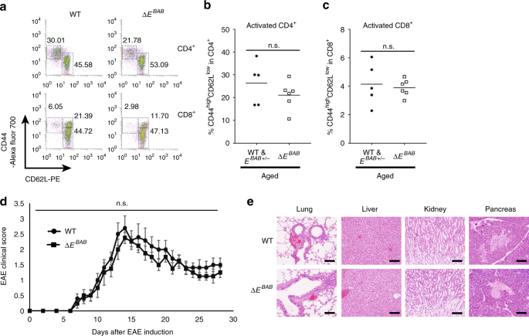Fig. 8 ΔEBABmice do not show any autoimmune phenotype.aFlow cytometric analysis of CD62L versus CD44 populations in CD4+or CD8+splenic T cell. The number in the plot is representative percentage of each gate. For CD4+T cells, gates indicate activated (CD44highCD62Llow) and naïve (CD44lowCD62Lhigh) populations. For CD8+T cells, activated effector memory (CD44highCD62Llow), activated central memory (CD44highCD62Lhigh) and naïve (CD44lowCD62Lhigh) populations are gated. Data are representative of four independent experiments (n= 5 for WT andEBAB+/−mice,n= 6 for ΔEBABmice from WT &EBAB+/−–ΔEBABlittermate pairs and trios, 30–34 weeks old).b,cActivated CD4+(b) and CD8+(c) proportions of aged mice. Data are pooled from four independent experiments (n= 5 for WT andEBAB+/−mice,n= 6 for ΔEBABmice from WT andEBAB+/−–ΔEBABlittermate pairs and trios, 30–34 weeks old).dThe mean (±s.e.m.) clinical scores at the days after EAE was induced in WT (control) (n= 10) and ΔEBABmice (n= 8). The incidence of EAE: control 10/10, ΔEBAB8/8. No data point showed statistically significant difference between WT and ΔEBAB(i.e., unpaired two-tailed Student’sttestP≥ 0.05).eRepresentative pictures for Hematoxylin and Eosin staining for the lung, liver, kidney, and pancreas of two independent experiments (n= 2 WT andEBAB+/−–ΔEBABlittermate pairs, 30–31 weeks old). The scale bars represent 100 μm. Each symbol in (b,c) represents an individual mouse; small horizontal lines indicate the mean. n.s. not significant (P≥ 0.05) (unpaired two-tailed Student’sttest) 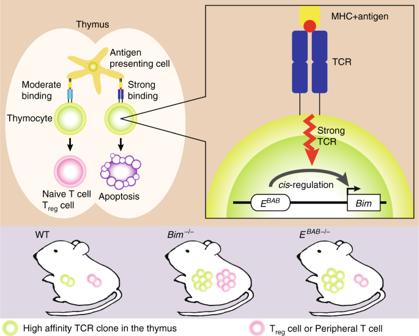Fig. 9 Graphical summary.EBABplays a role in inducing TCR signal-dependent apoptosis to eliminate high affinity TCR clones in the thymus while dispensable forBim-dependent peripheral T cell tolerance Mice were then injected with 200 ng of Pertussis Toxin (Calbiochem) intraperitoneally at day 0 and day 2 after EAE induction. The clinical scores were assessed as follows: (1) flaccid tail, (2) impaired righting reflex and/or gait, (3) partial hind limb paralysis, (4) total hind limb paralysis, and (5) total hind limb paralysis with partial forelimb paralysis. Statistics The sample size was chosen as follows. First, the number of animals was minimized as much as possible in light of animal ethics. Second, against effect size estimated in each experiment, ≥80–90% power was favored. Third, in most cases, n = 5 was set as a threshold according to the previous report [55] . These three criterion functioned to determine the sample size as n = 5–8 in most experiments. Moreover, dot-plot/box plot representation of data provided insights into how the samples were distributed, and thus into the extent of difference of two groups. This, in the specific cases, led us to conclude that relatively small number of animals (i.e., less than five animals) was enough to support our conclusion. According to the observed differences, our sample size appeared to be appropriate to meet≥80–90% power. In addition, dot-plot/box plot representation of data was useful to estimate sample distribution. Clearly abnormal distribution was not observed in our experiments, further supporting that our statistical tests were appropriate. Significant differences between two groups were examined using one or two-tailed, unpaired t test, or Mann–Whitney U test. One-tailed test was chosen when we had hypothesis and/or previous knowledge regarding direction of changes (e.g., increased or decreased) in experiments. Reporting summary Further information on research design is available in the Nature Research Reporting Summary linked to this article.